Discriminating cellular heterogeneity using microwell-based RNA cytometry Discriminating cellular heterogeneity is important for understanding cellular physiology. However, it is limited by the technical difficulties of single-cell measurements. Here we develop a two-stage system to determine cellular heterogeneity. In the first stage, we perform multiplex single-cell RNA cytometry in a microwell array containing over 60,000 reaction chambers. In the second stage, we use the RNA cytometry data to determine cellular heterogeneity by providing a heterogeneity likelihood score (HLS). Moreover, we use Monte-Carlo simulation and RNA cytometry data to calculate the minimum number of cells required for detecting heterogeneity. We apply this system to characterize the RNA distributions of ageing-related genes in a highly purified mouse haematopoietic stem cell population. We identify genes that reveal novel heterogeneity of these cells. We also show that changes in expression of genes such as Birc6 during ageing can be attributed to the shift of relative portions of cells in the high-expressing subgroup versus low-expressing subgroup. Determining whether a cell population is heterogeneous, whether it consists of distinct subpopulations, is important for understanding cellular physiology and identifying therapeutic targets. To effectively detect heterogeneity, high-throughput analysis of individual cells is required. A current technology that provides such an analysis, flow cytometry, has revolutionized our understanding of how cells are regulated and operate. For example, in immunology and haematology, flow cytometry has led to the identification of stem cells and the process of haematopoiesis, the development of antiretroviral agents for treating HIV infection and improvements in bone marrow transplantation to treat blood diseases, such as myelodysplastic syndrome [1] . While flow cytometry is effective, it is limited by the availability of antibodies. Only a minority of known human genes have commercially available antibodies. Flow cytometry is also difficult to perform when the distinguishing features of subpopulations are molecules inside the cells rather than on the surface of cells. Detecting intracellular features such as specific mRNA molecules does not require antibodies and possesses enormous potential because it can exploit the genomics and microarray data and provides new opportunities to define novel subpopulations of cells. To uncover gene markers that fractionate a cell population, single-cell mRNA abundance measurements are required. Developments in florescent in-situ hybridization (FISH) techniques have demonstrated the ability to count individual mRNAs within single cells [2] . However, single RNA molecule detection through FISH requires optimized cell fixation protocols that are not universally applicable to all tissues and cell types. In addition, tens of probes per RNA molecule need to be designed to generate a detectable signal. These requirements limit the samples and cell types that can be used and the number of RNA molecules that can be detected in each cell [3] . A much simpler technique for mRNA quantification that has a large dynamic range and is amenable to high throughput analysis is reverse transcription polymerase chain reaction, RT–PCR [3] . Miniaturization is an effective way for increasing the analysis throughput of RT–PCR and for reducing the signal dilution. A variety of microfluidic systems have been developed to compartmentalize PCR mixtures into nano to femtolitre reaction volumes, including valve-actuated microfluidic systems [4] , microdroplets of water-in-oil emulsions [5] and microwell arrays [6] . However, because of the complexity of handling single cells and multi-step RT–PCR protocols, the vast majority of microfluidic techniques have been limited to analysing less than 100 single cells per run. Measuring the mRNA levels in less than 100 single cells would not be sufficient. mRNA detection with single-cell resolution suffers from high levels of variability [7] . This variability is at least partially due to biophysical reasons such as, 1 inherent random variability from the Brownian motion of low abundance intracellular reactant molecules [8] ; 2 intercellular mRNA time point variability (expression burst cycles) within clonal populations [9] ; and technical reasons such as the measurement noise associated with diluting the low amount of target mRNA from a single cell (~10 pg) into the microliter plate well volume [10] (3–50 μl). This variability in the RNA levels, of single cells, has been reported and approximated through a log-normal distribution [11] . This implies that subgroups of cells with different RNA expression characteristics would exhibit log-normal distributions with varying mean, s.d. and proportion parameters. Hence, to detect whether a cell sample is heterogeneous, the number of log-normal components that make up the sample expression distribution have to be detected. In many cases, to detect the number of components with a high statistical power, thousands to tens of thousands of single-cell measurements are required ( Fig. 1 ). Commonly, most gene expression levels vary in the range of 2–4 times the basal level, depending on the cell type and/or cell state. In addition, many important subpopulations may be composed of rare cells (that is, with frequencies of less than 5% of the entire cell population). Thus, being able to analyse significantly more cells is critical for the discovery of rare subpopulations with medium to low mRNA differences. 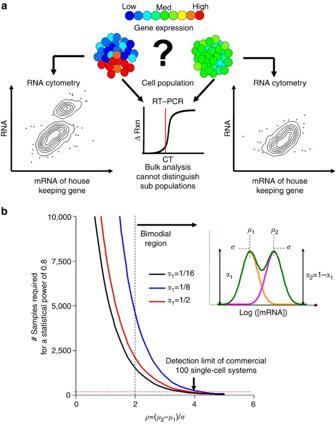Figure 1: Multiplex single-cell RNA analysis can discriminate cell population heterogeneity. (a) Conventional bulk analysis using reverse transcriptase polymerase chain reaction (RT–PCR) cannot discriminate individual cells within a population. By separating a whole population of cells into single-cell reactions, RNA levels in each cells can be determined. This can reveal subpopulations of cells based on RNA abundance. (b) Genes expressed in single cells generate mRNA abundance that follow random log-normal distributions. To be able to distinguish with a statistical power of >0.8 between different subpopulations of cells, the log-mRNA distribution for the gene of interest has to be accurately measured to correctly detect the number of normal (gaussian) components that make up the distribution. The minimum sample size required for correct subpopulation detection depends on the separation of the components (μ2−μ1), their s.d.σand frequency parameterα1. The inset shows a two-component distribution (green line) and the key parameters that characterize each Gaussian component (yellow and purple lines). Please note that the horizontal axis represents the logarithm of the mRNA abundance. Figure 1: Multiplex single-cell RNA analysis can discriminate cell population heterogeneity. ( a ) Conventional bulk analysis using reverse transcriptase polymerase chain reaction (RT–PCR) cannot discriminate individual cells within a population. By separating a whole population of cells into single-cell reactions, RNA levels in each cells can be determined. This can reveal subpopulations of cells based on RNA abundance. ( b ) Genes expressed in single cells generate mRNA abundance that follow random log-normal distributions. To be able to distinguish with a statistical power of >0.8 between different subpopulations of cells, the log-mRNA distribution for the gene of interest has to be accurately measured to correctly detect the number of normal (gaussian) components that make up the distribution. The minimum sample size required for correct subpopulation detection depends on the separation of the components ( μ 2 − μ 1 ), their s.d. σ and frequency parameter α 1 . The inset shows a two-component distribution (green line) and the key parameters that characterize each Gaussian component (yellow and purple lines). Please note that the horizontal axis represents the logarithm of the mRNA abundance. Full size image An important place to look for heterogeneity is within the population of hematopoietic stem cells (HSCs). Although HSCs have been isolated with high purity [12] , it has been shown that young and old HSCs exhibit heterogeneity in function when transplanted into irradiated recipients [13] , [14] , [15] , [16] , [17] , [18] , [19] , [20] . Previous studies suggest that age-dependent alterations in gene expression of HSCs modulate their differentiation potential and may contribute to age-related immune system decline [21] . Age-dependent gene expression changes in the entire HSC population have been previously identified [21] . However, it has been recently proposed that these changes may not be due to epigenetic changes within the HSC population, but instead it may be caused by the difference in proliferation of distinct HSC subpopulations with relatively constant gene expression signatures [18] , [22] . This implies a new mechanism of HSC ageing that relies on competition between different subpopulations. Old HSCs exhibit myeloid lineage bias more frequently than young HSCs. In addition, there is evidence that myeloid-biased HSCs proliferate faster [17] . On the basis of this functional evidence of HSC heterogeneity, here we look for gene markers that can reveal novel subgroups of HSCs. Thus, we ask (1) can we identify mRNA abundance markers that clearly distinguish unknown subgroups within a highly pure HSC population? (2) Are these markers associated with HSC ageing and if so, do the relative group sizes correlate with ageing as a potential indication of subpopulation competition? This second question has clinical implications, because, as human HSCs age, they become more susceptible to certain myeloproliferative disease, such as acute myeloid leukaemia. Identifying the source of this lineage bias in ageing HSCs may point to therapeutic targets for treating age-associated myeloproliferative disorders. In this study, we develop a novel two-step system for heterogeneity detection. In the first step, we apply microwell RNA cytometry, which we have optimized to simultaneously perform thousands of multiplex single-cell RT–PCR assays. In the second step, using the RNA cytometry data, we estimate subpopulation distribution parameters to determine the number of single-cell measurements that need to be aggregated to overcome RNA variability and reveal the underlying population components. Also in Step 2, we aggregate and analyse the RNA cytometry results to generate a HLS that indicates the statistical significance of the uncovered sub-populations. Finally we apply this technique to determine the heterogeneity of highly purified hematopoietic stem cell populations. We have identified novel gene markers that split the HSC population in a bi-modal manner and provide novel insight into HSC ageing. Microwell RNA cytometry For Step 1, we perform RNA cytometry ( Supplementary Fig. 1 ) to measure specifically the mRNA abundance in thousands of single cells. We start by evaluating the feasibility of generating end point fluorescent signals that can semi-quantitatively reflect the initial amount of nucleic acid target. The advantage of using end point fluorescent is that it significantly reduces photobleaching as compared with real-time analysis that requires exciting the fluorophores during every cycle of the PCR reaction. Photobleaching is an important concern when the reaction volume is small (~20 pl). In addition, it considerably simplifies the required setup for performing RNA cytometry. It has been previously demonstrated [23] that by reducing the amplification reaction volume the PCR amplification slope (and thus the reaction efficiency) is decreased, probably due to the high surface to volume ratio. As a consequence, the log-linear range of the PCR reaction is prolonged, even beyond 40 cycles [23] . Taking advantage of this phenomenon [24] , [25] , [26] , we performed on-chip tests by amplifying genomic DNA from the nanog promoter region. Targeting the nanog promoter region within the nucleus of a live cell would also determine how the proteins present in the cell affect the PCR reaction. To obtain a range of cell numbers per well, we loaded the array with a high concentration of cells. After loading the cells and before the PCR, we manually counted and recorded the number of cells in each well. The data suggest a log-linear trend between the well intensity and the number of cells per well ( Fig. 2 ). Note that the initial background fluorescence from the DNA before PCR has been subtracted, and only pixels corresponding to the free in solution fluorescence were used to calculate the mean intensity. Thus, all pixels that correspond to the fluorescent intensity from the cells are discarded. The background fluorescence was quantified from the empty wells after 40 cycles of PCR. From previous mRNA counting experiments [27] , single-cell mRNA expression has been shown to vary substantially, in certain cases such as PDR5 from 0 to 40 mRNA transcripts per single cell. Thus, we verified if the 40 cycle end point fluorescence log-linear trend is consistent over a wider range of initial template numbers. For that purpose, we spiked in known amounts of pAW109 RNA transcripts and performed microwell RT–PCR for 40 cycles. RT–PCR was performed as explained in the ‘RT–PCR amplification’ section. From Fig. 2e , we can see that the end point fluorescent signals scale linearly with the logarithm of the initial RNA concentration. Increasing the cycle number beyond the 40 cycles is not beneficial because that increases the number of dried 20 pl microwells around the edge, while decreasing the 40 cycles reduces the overall fluorescent intensity and the signal to noise ratio. 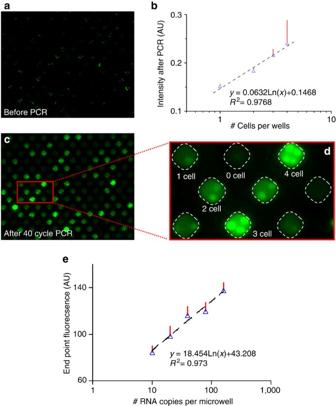Figure 2: The end point fluorescence of the ~20 pl microwell PCR reaction is proportional to the logarithm of the initial amount of target DNA (that is, log-linear). (a) A representative image of a 15,000-well array before PCR. Scale bar, 40 μm. (b) The clear log-linear trend between well intensity at cycle 40, and the number of cells per well after amplifying the promoter region of theNanoggene suggests that the well intensity is a semi-quantitative indicator of the initial amount of target DNA. Error bars represent s.e. (n=50 for 0–3 cells per well andn=4 for 4 cells per well). Note that the initial background fluorescence coming from the nuclear DNA before PCR has been subtracted, and the mean intensity is the signal from the free in-solution fluorescence. (c) Representative image from the microwell array after 40 cycles for PCR. Scale bar, 40 μm. (d) Magnified image of a representative region with wells containing, 0, 1, 2, 3 and 4 cells. The array was loaded with ~500 cell per μl in a total volume of 60 μl. The dashed lines represent the well boundaries. Note that all pixels that correspond to the fluorescent intensity from the cells are discarded from the quantification, thus only the area corresponding to the free, in-solution fluorescence is quantified. Scale bar, 20 μm. (e) Log-linear relation between end point fluorescence (40 cycles) and starting number of spiked in pAW109 RNA templates. Error bars represent s.e. (n=20). Figure 2: The end point fluorescence of the ~20 pl microwell PCR reaction is proportional to the logarithm of the initial amount of target DNA (that is, log-linear). ( a ) A representative image of a 15,000-well array before PCR. Scale bar, 40 μm. ( b ) The clear log-linear trend between well intensity at cycle 40, and the number of cells per well after amplifying the promoter region of the Nanog gene suggests that the well intensity is a semi-quantitative indicator of the initial amount of target DNA. Error bars represent s.e. ( n =50 for 0–3 cells per well and n =4 for 4 cells per well). Note that the initial background fluorescence coming from the nuclear DNA before PCR has been subtracted, and the mean intensity is the signal from the free in-solution fluorescence. ( c ) Representative image from the microwell array after 40 cycles for PCR. Scale bar, 40 μm. ( d ) Magnified image of a representative region with wells containing, 0, 1, 2, 3 and 4 cells. The array was loaded with ~500 cell per μl in a total volume of 60 μl. The dashed lines represent the well boundaries. Note that all pixels that correspond to the fluorescent intensity from the cells are discarded from the quantification, thus only the area corresponding to the free, in-solution fluorescence is quantified. Scale bar, 20 μm. ( e ) Log-linear relation between end point fluorescence (40 cycles) and starting number of spiked in pAW109 RNA templates. Error bars represent s.e. ( n =20). Full size image An essential aspect of the RNA cytometry process is the ability to load single cells in microwells. By controlling the total number of loaded cells, we can optimize for single-cell trapping. In a typical setup, 120 μl of cell suspension is placed over the microwell array and centrifuged to randomly distribute and settle the cells across the array. Supplementary Fig. 1 shows a detailed schematic outline of the microwell chip array operation. To establish the ideal concentration, we calculated the relationship between the concentration of cells (cells per μl) with the percentage of wells consisting of zero, one or more than one cell per well using a probability model. This model is validated with our experimental data ( Fig. 3 ). Depending on the frequency and the gene expression difference of the subpopulation of interest, a range of operating concentrations was determined. We chose an operational range 10 and 110 cells per μl to fill 4–33% wells with single cells and exclude multiple cell per well trapping (between 0.06 and 6%). 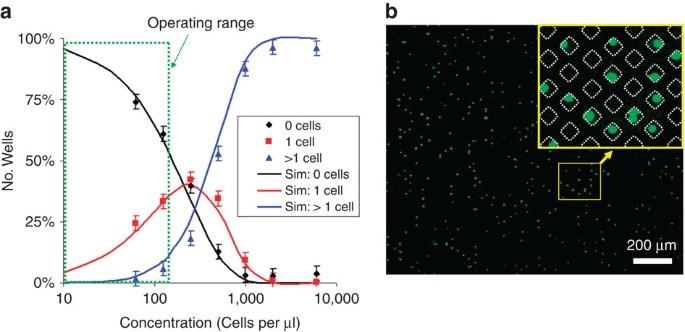Figure 3: Single-cell trapping analysis. (a) The graph illustrates the relation between the concentration of cells (cells per μl) and the fraction of wells containing zero, single or multiple cells. The total loading volume for all concentrations was 60 μl. The solid lines represent calculated results, the points represent experimental data and error bars represent the standard error (n=3). The dotted box labelled ‘Operating Range’ marks the ideal range of operation that guarantees a low number of multiple cell trappings (<9%). The exact concentration can be chosen by selecting the maximum number of allowed multiple cell trappings. For example, if a full array of 60,000 microwells is filled with ~20,000 cells then ~15,000 wells will be filled with single cells and ~3,000 wells will contain two or more cells. This means that roughly 5% of all the wells have two or more cells. For applications where the number of wells with two or more cells has to be reduced, loading ~2,400 cells into a 60,000 microwell array would result in ~0.068% of all the wells having two or more cells. (b) Representative fluorescence micrograph of a loaded microwell array. The inset shows magnified image of a region of the chip with 13 single-cell wells and one two-cell well. The wells are outlined with the white dotted lines. Scale bar, 200 μm. Figure 3: Single-cell trapping analysis. ( a ) The graph illustrates the relation between the concentration of cells (cells per μl) and the fraction of wells containing zero, single or multiple cells. The total loading volume for all concentrations was 60 μl. The solid lines represent calculated results, the points represent experimental data and error bars represent the standard error ( n =3). The dotted box labelled ‘Operating Range’ marks the ideal range of operation that guarantees a low number of multiple cell trappings (<9%). The exact concentration can be chosen by selecting the maximum number of allowed multiple cell trappings. For example, if a full array of 60,000 microwells is filled with ~20,000 cells then ~15,000 wells will be filled with single cells and ~3,000 wells will contain two or more cells. This means that roughly 5% of all the wells have two or more cells. For applications where the number of wells with two or more cells has to be reduced, loading ~2,400 cells into a 60,000 microwell array would result in ~0.068% of all the wells having two or more cells. ( b ) Representative fluorescence micrograph of a loaded microwell array. The inset shows magnified image of a region of the chip with 13 single-cell wells and one two-cell well. The wells are outlined with the white dotted lines. Scale bar, 200 μm. Full size image Next we demonstrate that RNA cytometry can be used to measure single-cell gene expression. We measured the expression level of glyceraldehyde 3-phosphate dehydrogenase (GapDH), in the cell line BB88: ATCC TIB-55. Single cells were randomly sedimented into a 20 pl microwell array, such that most wells contained either a single cell or no cell ( Fig. 3 ). After thermally cycling the array, the GapDH fluorescent signal was captured by fluorescently imaging the array ( Fig. 4 ). The mean intensity was calculated for each microwell. This information was plotted in a histogram ( Fig. 5 ), revealing that a higher intensity distribution was formed after the thermal cycling, suggesting the existence of microwells with a high abundance of mRNA. Eliminating the reverse transcriptase from the reaction disabled the formation of this higher intensity distribution ( Fig. 6a ). To distinguish between high-intensity and low-intensity wells, we defined a threshold fluorescence f tr = μ norm +3 σ ( Fig. 5b ), where μ norm and σ represent the mean and the s.d., respectively, of a gaussian fit over the low well intensity histogram. Thus, low-intensity wells are defined as having a mean fluorescent intensity of less than f tr . The low fluorescent intensity is mainly due to wells that did not contain any cells. Thus, in the case where all the cells contain the target mRNA and there is no inhibition of the RT–PCR reaction, the number of high-intensity wells will be approximately equal to the total number of cells loaded. Within the microwell array, the low-intensity wells are used as a normalization control. All intensities are normalized to the mean of the low intensity wells after the RT–PCR reaction. These wells represent the background fluorescent intensity ( Fig. 5b ). For clarity of data display, the low-intensity well data points are removed from the histograms and scatter plots shown in this article, unless specifically noted. 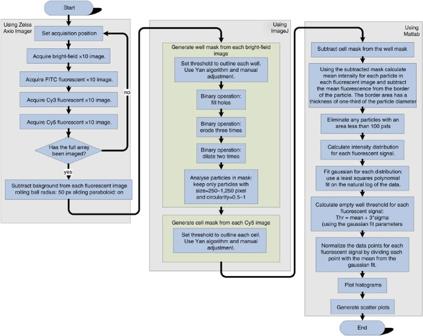Figure 4: Signal acquisition, processing and normalization. The process starts by scanning the microwell array with an automated epifluorescent microscope system. The whole array is scanned at × 10 and saved onto 108 1,388 × 1,040 tiff images. With the use of custom scripts in ImageJ, the global background is subtracted from each fluorescent image and the location of each microwell is established by thersholding. The Cy5 images are used to locate each cell within the microwell so that the pixels from that cells are removed from the intensity analysis. A custom MatLAB script is used to calculate the mean florescence of the free solution in each microwell. Local normalization is performed by subtracting the mean fluorescence surrounding the well (within a radius of 1/3 the size of the microwell). This minimizes intensity variations that can be due to uneven fluorescent excitation. The Cy5 quantification represents the amplification ofActinB, so it is used to calculate the threshold fluorescence and eliminate the wells without cells from the plots. The mean intensity of the empty wells is used to normalize the fluorescence signal in each channel. All plotting of the density scatter plots was done using custom scripts within MatLAB. Figure 4: Signal acquisition, processing and normalization. The process starts by scanning the microwell array with an automated epifluorescent microscope system. The whole array is scanned at × 10 and saved onto 108 1,388 × 1,040 tiff images. With the use of custom scripts in ImageJ, the global background is subtracted from each fluorescent image and the location of each microwell is established by thersholding. The Cy5 images are used to locate each cell within the microwell so that the pixels from that cells are removed from the intensity analysis. A custom MatLAB script is used to calculate the mean florescence of the free solution in each microwell. Local normalization is performed by subtracting the mean fluorescence surrounding the well (within a radius of 1/3 the size of the microwell). This minimizes intensity variations that can be due to uneven fluorescent excitation. The Cy5 quantification represents the amplification of ActinB , so it is used to calculate the threshold fluorescence and eliminate the wells without cells from the plots. The mean intensity of the empty wells is used to normalize the fluorescence signal in each channel. All plotting of the density scatter plots was done using custom scripts within MatLAB. 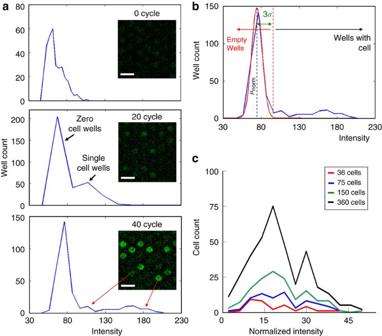Figure 5: Subpopulation discrimination based on hundreds of single-cell RT–PCR reactions. (a) High throughput single-cell gene expression analysis was performed by loading the microwell array with BB88 cells. A representative florescent micrograph and the well intensity histogram at cycles 0, 20 and 40 are shown. The histograms include the intensity of all the wells (including empty wells and wells containing single cells). Scale bars, 40 μm. (b) The fluorescent threshold is calculated to eliminate the empty low-intensity wells and normalize the fluorescent intensity signals of the higher fluorescing wells. Note that the empty wells’ fluorescence levels remained approximately constant and similar to the background throughout the 40 amplification cycles. In addition, the empty wells are approximately 3- to 10-fold more numerous than the single-cell wells. This characteristic was harnessed to calculate the low intensity well threshold using a linear regression gaussian fit and then setting the threshold (ftr) atμnorm+3σ, whereμnormandσrepresent the mean and the s.d., respectively. (c) Histograms of the single-cell well intensities of the RT–PCR reactions of mouse peripheral blood mononuclear cells (PBMCs) cells, which are known to be heterogeneous (bi-modal) for Mac-1 expression. The well intensities are calculated as the ratio of the mean intensity of the free solution fluorescence within the well versus the mean empty well intensity. As predicted inFig. 1ba statistically significant number (~360) of single cells is required for the histogram distribution to clearly show the presence of two distinct cell populations in the mixture (P<0.1,P-value calculated as shown inSupplementary Fig. 9). Full size image Figure 5: Subpopulation discrimination based on hundreds of single-cell RT–PCR reactions. ( a ) High throughput single-cell gene expression analysis was performed by loading the microwell array with BB88 cells. A representative florescent micrograph and the well intensity histogram at cycles 0, 20 and 40 are shown. The histograms include the intensity of all the wells (including empty wells and wells containing single cells). Scale bars, 40 μm. ( b ) The fluorescent threshold is calculated to eliminate the empty low-intensity wells and normalize the fluorescent intensity signals of the higher fluorescing wells. Note that the empty wells’ fluorescence levels remained approximately constant and similar to the background throughout the 40 amplification cycles. In addition, the empty wells are approximately 3- to 10-fold more numerous than the single-cell wells. This characteristic was harnessed to calculate the low intensity well threshold using a linear regression gaussian fit and then setting the threshold ( f tr ) at μ norm +3σ, where μ norm and σ represent the mean and the s.d., respectively. ( c ) Histograms of the single-cell well intensities of the RT–PCR reactions of mouse peripheral blood mononuclear cells (PBMCs) cells, which are known to be heterogeneous (bi-modal) for Mac-1 expression. The well intensities are calculated as the ratio of the mean intensity of the free solution fluorescence within the well versus the mean empty well intensity. As predicted in Fig. 1b a statistically significant number (~360) of single cells is required for the histogram distribution to clearly show the presence of two distinct cell populations in the mixture ( P <0.1, P -value calculated as shown in Supplementary Fig. 9 ). 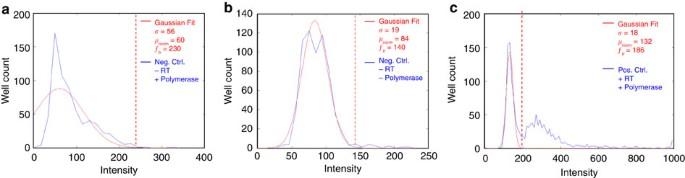Figure 6: Verification of specific mRNA amplification. (a) Single-cell RT–PCR ofActBmRNA in BB88 cells with reverse transcription omitted and only PCR thermocycling performed. A histogram of the well intensities showing no amplification signal over the empty well thresholdftr(well intensities overftrrepresented by the red dotted line). This demonstrates that DNA is not amplified. (b) Single-cell RT–PCR ofActBmRNA in BB88 cells after removing the RT and polymerase enzymes from the reaction mix. A histogram of the well intensities showing no amplification signal over the empty well thresholdftr(well intensities overftrrepresented by the red dotted line). No DNA or RNA is amplified. (c) Single-cell RT–PCR ofActBmRNA in BB88 cells, positive control where RT and polymerase enzymes are included and the standard thermocycling protocol is performed. Histogram of the well intensities showing a clear presence of amplification signal over the empty well thresholdftr(signal above the red dotted line). Note all reactions are done using the CellsDirect, Invitrogen kit as described in the Methods, RT–PCR Amplification section.ftrindicates threshold fluorescence;μnorm, mean; andσ, s.d. Full size image Figure 6: Verification of specific mRNA amplification. ( a ) Single-cell RT–PCR of ActB mRNA in BB88 cells with reverse transcription omitted and only PCR thermocycling performed. A histogram of the well intensities showing no amplification signal over the empty well threshold f tr (well intensities over f tr represented by the red dotted line). This demonstrates that DNA is not amplified. ( b ) Single-cell RT–PCR of ActB mRNA in BB88 cells after removing the RT and polymerase enzymes from the reaction mix. A histogram of the well intensities showing no amplification signal over the empty well threshold f tr (well intensities over f tr represented by the red dotted line). No DNA or RNA is amplified. ( c ) Single-cell RT–PCR of ActB mRNA in BB88 cells, positive control where RT and polymerase enzymes are included and the standard thermocycling protocol is performed. Histogram of the well intensities showing a clear presence of amplification signal over the empty well threshold f tr (signal above the red dotted line). Note all reactions are done using the CellsDirect, Invitrogen kit as described in the Methods, RT–PCR Amplification section. f tr indicates threshold fluorescence; μ norm , mean; and σ , s.d. Full size image Detecting subpopulations with RNA cytometry Recently, microwell array RT–PCR [28] was demonstrated to exhibit a high level of specificity when assaying for a single gene. However, to examine cellular heterogeneity we have to distinguish whether a low PCR signal is due to RT–PCR failure or truly represents a low gene expression. Thus, it is necessary to include a technical control for the RT–PCR reaction, by measuring at least one housekeeping mRNA in conjunction with the gene of interest ( Supplementary Fig. 2 ). From Supplementary Fig. 2 we can see that if a standard normalization is done directly using only a single gene, wells with low expressing cells have a similar intensity to the empty or background intensity wells, making them indistinguishable. In contrast, if a housekeeping gene is used as an indicator of a successful RT–PCR reaction and a non-empty well, then the low mRNA-expressing cells are detected and shown to form a subgroup. The measurement of two different mRNAs per cell requires performing a multiplexed RT–PCR reaction in each microwell. The multiplexed reactions were achieved with multi-colour (FAM and Cy5 labelled) Taqman probes and primers for the genes of interest and for the housekeeping gene β-actin ( ActB ) (see Supplementary Fig. 3 ). Using the β-actin housekeeping gene and the end point fluorescence measurements, we confirm the capability of RNA cytometry to detect subpopulations. As a demonstration, we probe known subpopulations within mouse peripheral blood mononuclear cells. Using peripheral blood mononuclear cells from 5-week-old C57Bl/6 mice, we look for the heterogeneous (bimodal) expression of integrin alpha M (Itgam) also known as macrophage-1 antigen (Mac-1). The results show a distribution of two subgroups of cells, with low and high Mac-1 mRNA abundance ( Fig. 5c ). Using least-squares fit of multiple-gauss peaks, we could estimate the relative sizes ( Supplementary Fig. 4 ) of the Mac-1 low (83.7%) and Mac-1 high (16.3%) populations. These results were verified using flow cytometry analysis of Mac-1 surface expression revealing that 17.1% of the cells were indeed Mac-1 high ( Supplementary Fig. 4B ). In addition, we have shown a known variation currently used in HSC purification ( Supplementary Fig. 4C ). Statistical confirmation of heterogeneity Next in Step 2, using the RNA cytometry data from Step 1 we estimate the minimum number of cells that have to be measured to be certain that we would able to detect any heterogeneity. To confirm whether a cell sample is heterogeneous based on a specific RNA (that is, gene), the number of log-normal components that make up that sample’s distribution has to be detected. Detecting the number of log-normal (gaussian distribution on a log(mRNA) scale) components with a high statistical power (>0.8) requires the aggregation of a sufficiently large number of single-cell measurements. On the basis of Monte Carlo simulations ( Fig. 1b ), the minimum number of cells required is a function of the minimum expected separation of the prospective subgroups ( μ 2 − μ 1 ), their s.d. ( σ of the log-normal distribution) and the minimum frequency α 1 . In practice, these parameters are not known a priori . However, from the RNA cytometry data (Step 1) we can estimate certain minimum separation limits. For example, from the Mac-1 experiments ( Fig. 5 ) we can estimate that the mixture contains two gaussian components with a mean separation ( μ 2 − μ 1 ) of ~1.92 fold μ 1 and a mean normalized s.d. of ~0.298. Thus, from Fig. 1b we can see that between 359 ( α 1 =0.5) and 507 ( α 1 =0.125) single-cell measurements would be required to correctly detect the sample heterogeneity. The two-peak distribution became apparent ( P <0.1, P -value calculated as shown in Supplementary Fig. 9 ) after aggregating more than 360 single cells ( Fig. 5c ). This verifies the Monte Carlo simulations ( Fig. 1b ). As an initial example, for HSC heterogeneity detection, we are interested in a mean expression difference of at least 2.5-fold, a minimum frequency α 1 of 12% and in the case of σ we assume that the normalized s.d. of the subpopulations we would like to detect within our genes of interest is less than or equal to the macrophage antigen-1 high population ( Supplementary Fig. 4 ), 0.142. This results in ( μ 2 − μ 1 )/σ ratio of Log (2.5)/0.142≈2.8, thus we should measure ~730 single cells to uncover subgroups with such a separation. Any subgroups with a larger separation [( μ 2 −μ 1 )/σ>2.8 or α 1 >12%] should be clearly evident after measuring 730 single cells. Next, we calculate if the RNA distribution measured with the RNA cytometry from step 1 is really heterogeneous. To do this, we calculate the HLS. This score is calculated based on the StepMiner algorithm and represents the probability that the distribution has more than one component (that is, it is heterogeneous). More established methods to estimate the existence of more than one component include Gaussian mixture modelling and goodness-of-fit criteria, such as BIC or ICL, to determine the number of Gaussian components (subpopulations). To confirm our HLS-based approach, we performed a head-to-head comparison between our StepMiner based method and a Gaussian mixture modelling approach. The Gaussian mixture model computation was done using ‘mixtools’ R package. We first used a kernel density estimation algorithm. Then we sampled 500 points from the PDFs of the fluorescence intensities. We employed an EM algorithm to estimate the gaussian mixture model. The results are consistent with those from StepMiner for all the genes except Dntt (see Supplementary Table 1 ). For Dntt , the EM algorithm identified two components while Log-Likelihood and BIC identified a single component best fit. Thus, fitting more than one component to Dntt could be considered overfitting. We show that for subpopulation identification and/or confirmation, the HLS calculations are consistent with other well-established statistical procedures. Probing for HSC heterogeneity To demonstrate the 2-stage heterogeneity detections system, we measured the mRNA distribution in highly purified ( Supplementary Fig. 5 ) primary HSCs from 2-month-old C57Bl/6 mice. To look for genes that can reveal a heterogeneous expression within the HSC population, we focus on ageing-related genes. We hypothesize that genes whose expression changes significantly with ageing are good candidates to split HSCs into a low- and high-expressing group. As the mouse ages, the increase in the average gene expression seen in the HSC population may be attributable to an increase in the relative size of a high-expressing subpopulation. On the basis of microarray analysis [21] of purified bulk HSCs, we selected five genes whose expression changes the most with ageing ( Table 1 ). In addition, based on previous studies [15] , [16] , [19] , we also included the age-related gene Slamf1 . Furthermore, we included CD41 (Itga2b) as a likely candidate for separating the HSC population. CD41 has been shown to be differentially expressed in HSCs [29] from newborn mice. All the microwell RT–PCR assays use exon-spanning primers to prevent amplification from genomic DNA. The fluorescent signals from each mRNA were normalized and plotted onto density scatter plots ( Fig. 7 ). Most of the age-related genes we examined exhibited a homogeneous distribution of mRNA content ( Fig. 7b and Supplementary Figs 6 and 7 ). Slamf1 and Itga2b showed a separation of the HSC population into low and high mRNA abundance groups ( Fig. 7a,c ). In addition, Birc6 showed a clear bimodal separation of the highly-pure FACS-sorted HSCs ( Supplementary Fig. 5 ) from the young mice into low- and high-expressing groups ( Fig. 8a ). The Birc6 bimodal separation was verified using a recently developed technique of mRNA in-situ hybridization ( Supplementary Fig. 8 ). Table 1 Gene assays used. 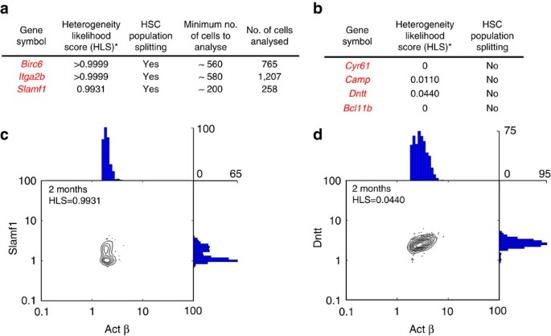Figure 7: Discriminating novel subgroups within purified haematopoietic stem cells (HSCs) from young (2 months old) mice. (a) List of the three genes candidates that resulted in population splitting. Because of the large number of single cells that were processed (on average ~2,000 single cells per gene) the separations exhibit a high HLS score with statistical significance (P<0.001). (b) List of the four gene candidates that did not split the young HSC population. (c) Signalling lymphocytic activation molecule (Slamf1) is a representative candidate gene that separates, in a bi-modal manner, the young HSC population into high and low expressers. (d) Deoxynucleotidyl transferase terminal (Dntt) on the other hand is a representative candidate gene that is differentially expressed in young and old HSCs but does not show a bimodal expression profile within the young HSC population. Full size table Figure 7: Discriminating novel subgroups within purified haematopoietic stem cells (HSCs) from young (2 months old) mice. ( a ) List of the three genes candidates that resulted in population splitting. Because of the large number of single cells that were processed (on average ~2,000 single cells per gene) the separations exhibit a high HLS score with statistical significance ( P <0.001). ( b ) List of the four gene candidates that did not split the young HSC population. ( c ) Signalling lymphocytic activation molecule ( Slamf1 ) is a representative candidate gene that separates, in a bi-modal manner, the young HSC population into high and low expressers. ( d ) Deoxynucleotidyl transferase terminal ( Dntt ) on the other hand is a representative candidate gene that is differentially expressed in young and old HSCs but does not show a bimodal expression profile within the young HSC population. 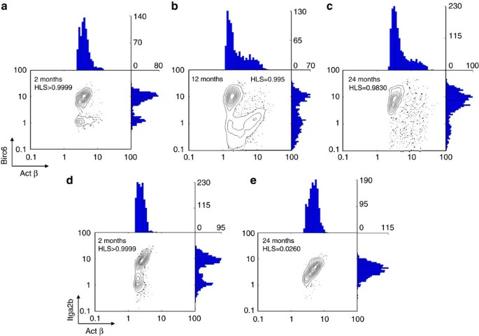Figure 8: Effect of ageing on the HSC subgroup proportions. (a–e) The effect of ageing on the expression profile ofBirc6andItga2bwas analysed by extracting HSC populations from 2 months, 1 year and 2 years old mice. Full size image Figure 8: Effect of ageing on the HSC subgroup proportions. ( a – e ) The effect of ageing on the expression profile of Birc6 and Itga2b was analysed by extracting HSC populations from 2 months, 1 year and 2 years old mice. Full size image We then asked whether the subpopulations separated by the Birc6 and Itga2b mRNA change with age. We examined HSCs from middle-aged (12-month-old) and old (24-month-old) mice. We found that the multi-component expression is substantially altered between the young mice as compared with the older mice for both Birc6 and Itga2b (CD41) ( Fig. 8a–e ). This alteration associated with ageing at least partially explains the overall gene expression change, previously detected with microarrays [21] . Recently, using FACS this alteration and reduction in heterogeneity in the CD41 expression profile between young and old mouse HSC were shown by Gekas and Graf [30] . They showed, at the protein level, that the number of CD41 high cells increases and dominates the overall population as the animal ages. Furthermore, CD41 expression was associated with myeloid-biased HSCs that increased with age. These findings are consistent with a model of clonal competition in which Birc6 -high expressing cells out-compete Birc6 -low cells over time, and the phenotype change previously identified [18] , [22] . Our calculations and results from Stage 1 and 2 show that hundreds to thousands of single cells need to be analysed to overcome single-cell variability and detect if a sample is heterogeneous. Thus, RNA cytometry, with its capability of up to 10,000 mutiplexed single-cell measurements can be an effective method for identifying markers that split cell populations based on RNA abundance. It can be applied to genes for which antibodies are not available. Effectively enabling heterogeneity detection based on genes that have previously been out of reach and the quantification of the tissue wide gene expression profiles with single-cell resolution. For heterogeneity detection, stage 2, minimum sample size and HLS calculations could be omitted. However, these indicators are useful to guide and confirm the search for cell subpopulations. In cases where no realistic numbers can be set for the minimum separation parameters ( μ 2 − μ 1 , σ , α 1 ), the maximum feasible number of single cells should be analysed. With 60,000 microwells, a single array can analyse over 10,000 single cells in one experiment. Our RNA cytometry method was designed to be feasible and accessible to common biology laboratories, because it does not require oxygen plasma bonding or other specialized equipment for loading and operation [28] . Hands-on operation of the microwell arrays requires less than 1 h and no specialized skills. Microwell arrays can be ordered from microfluidic device providers. An important part in the search for gene markers that can identify heterogeneity within seemingly pure cell populations is selecting a priori the likely gene candidates. For a non-biased approach, genome-wide bio-informatics algorithms can be used. MidREG analysis [31] for mutually exclusive genes is particularly suitable when looking for gene candidates that can split a population in a multi-modal manner. To reduce the need for selecting a priori the likely gene candidates more genes could be analysed simultaneously. With laser excitation, sharper band-pass filters and narrower emission fluorophores RNA cytometry can be extended to 12 or more simultaneous RNA targets. Moreover, with the help of a microarray printing robot and barcoded primers, microwell RT–PCR could be combined with high throughput RNA sequencing. This would reveal the full transcriptome of every single cell and eliminate the need for a priori gene candidate selection. However, the limitation of this approach could be that the maximum number of reads achievable with high throughput sequencing might not be sufficient to detect the low abundance mRNA. Identifying mRNA markers also allows for further characterization of cellular function. For example, the new subpopulation can be tracked or removed using the gene markers. In addition, direct functional analysis of RNA cytometry identified subpopulations can be achieved by generating fluorescent protein reporter cells, using the promoters of the identified gene markers. Thus, viable high- and low-expressing reporter cells can be sorted using FACS for in vitro and in vivo experimentation. Our experimental system detects cell subpopulations based on mRNA measurement. Heterogeneity in mRNA levels can be different from that in protein levels [32] , due to gene expression regulations such as mRNA modification and transportation, translation regulation, protein folding, modification, degradation and transportation. Thus, bimodality observed in mRNA levels does not necessarily translate into bimodality in protein level. For example, Slamf1 does not split HSCs at the protein level, while we detected bimodality in its mRNA level. It is possible that stochastic production or destruction of Slamf1 mRNA may have a role [33] . In our measurements of mouse HSCs, three of the seven measured ageing-related gene profiles ( Birc6 , Itga2b and Slamf1 ) showed heterogeneous (bi-modal) distributions. This provides new evidence of HSC heterogeneity, allowing for better understanding of HSC ageing and HSC regulation. Identifying subpopulations is not only critical for studying stem cell biology, tissue homeostasis and development, but it can also help to better understand the heterogeneity underlying cancer tissue [34] , [35] , [36] and allow for developing more effective and targeted anticancer therapies. Design and Fabrication of microwell arrays Using standard photolithography silicon masters, a microwell array (wells: 20 × 20 μm 2 and 50 μm deep) was fabricated. In brief, in this fabrication process, a mould was created using negative photoresist SU8-3010 (Microchem, Newton, MA, USA). The SU8-3010 was deposited on a clean silicon wafer using a spin coater (Brewer Science Spinner, Rolla, MO, USA). The photoresist was spread onto the wafer at 500 r.p.m. for 10 s and then ramped up to 1,000 r.p.m. at an acceleration of 300 r.p.m. per second. Once 1,000 r.p.m. was reached, the substrate was spun for 30 s to form a 25-micron layer. The wafer was then soft baked at 95 °C for 10 min. A second layer was spread onto the wafer at 500 r.p.m. for 10 s and then ramped up to 1,000 r.p.m. at an acceleration of 300 r.p.m. per second. Once 1,000 rpm was reached, the substrate was spun for 30 s to form a second 25-micron layer achieving a total height of 50 micrometres. The wafer was then soft baked at 95 °C for 10 min. After soft baking, the wafer was exposed for 30 s at 5.8 mW cm −2 using an OAI Hybralign Series 400 (Optical Associates, San Jose, CA, USA) mask aligner. The wafer was post-exposure baked for 1 min at 65 °C and 5 min at 95 °C. It was then allowed to cool to room temperature and developed in SU-8 Devloper (Microchem, Newton, MA, USA) for 4 min. PDMS was prepared according to the manufacturer’s instructions, degassed in a vacuum chamber for 30 min and spun coated at 1,000 r.p.m. 30 s onto the mould to form a 150-μm PDMS layer. PDMS was cured at 90 °C for 3 min on a hot plate and peeled off. For support, the PDMS microwell array was bonded on a 25 mm × 70 mm × 1 mm (VWR International, USA) microscope glass slide with the wells facing away from the slide. Bonding was done by exposing the PDMS and glass to 30 s of oxygen plasma treatment (Plasmod, Tegal Corp., Novato, CA, USA) and then placing them in conformal contact. Each microwell array contains an interlaced 250 × 250 grid of wells, so on a 10 × 10 mm footprint, there were 62,500 wells. Cell culture BB88 (ATCC TIB-55, Manassas VA, USA) mouse and HL60 (ATCC CCL-240, Manassas VA, USA) human cell lines were cultured in IMDM (Gibco Invitrogen, Carlsbad, CA, USA) supplemented with 10% fetal calf serum (FCS; Omega Scientific, Tarzana, CA, USA), 2 mM L -glutamine (Gibco Invitrogen), and 1 × Penicillin-Streptomycin (Gibco Invitrogen). The cell lines were maintained in 25 cm 2 canted-neck flasks (BD Falcon, BD Biosciences, San Diego, CA, USA) in 5% CO 2 at 37 °C and were split every 3 days to 1 × 10 5 cells per ml. Prospective isolation of haematopoietic stem cells Bone marrow cells were collected from 2-, 12- and 24-month-old C57Bl/6 male mice, and mononuclear cells were isolated using density gradient (Histopaque 1077, Sigma, St Louis, MO). Mononuclear cells were then purified using anti-CD117 microbeads (Milteny Biotec, Aubum, CA). Cells in the CD117-positive fraction were stained with monoclonal antbodies and sorted on FACSAria (BD Bioscience, San Jose, CA). The following monoclonal antibodies were purchased from eBioscience (San Diego, CA) and used: anti-CD34 (RAM34) conjugated to FITC (fluorescein isothiocyanate); anti-FL2/Flt3 (A2F10) conjugated to phycoerythrin (PE); anti-CD127/Il7ra (A7R34) conjugated to PE-Cy5; anti-CD4 (GK1.5), -CD8 (53-6.7), -B220 (RA3-6B2), -Ter119 (TER119), -Mac-1 (M1/70), and anti- Gr-1 (RB6-8C5) conjugated to PE-Cy7; anti-c-Kit (2B8) conjugated to APC-Alexa Fluor 750. Monoclonal antibody anti- Sca-1 (E13-161-7) was purified from a hybridoma and conjugated to Pacific Blue in the Weissman laboratory. Mice C57Bl/6 mice were used throughout this study. All mice were maintained in Stanford University’s Research Animal Facility, and all animal procedures were approved by the International Animal Care and Use Committee and Stanford University’s Administrative Panel on Laboratory Animal Care. Cell preparation and loading For loading the cells, a 3-mm high gasket was manually cut out of PDMS and place around the microwell array to form a well. Two hundred microlitres of PBS was added to the microwell array ( Supplementary Fig. 1 ). The array glass slide was placed on the 96-well plate lid and centrifuged (Beckman Coulter, Concord, MA, USA) at 3,000 r.p.m. for 5 min to completely wet the microwells. The PBS was then removed with a pipette. Depending on the assay, between 1,000 and 10,000 cells in 100 μl of PBS and 10% FCS were added within 1 min of removing the PBS. The array was then centrifuged (Beckman Coulter) at 4 °C 1,200 r.p.m. for 5 min. Single-cell loading was visually verified using a phase contrast culture microscope (Nikon Eclipse TS10) at × 10. The loaded cells were dehydrated by placing the array slide on an Eppendorf Mastercycler Gradient (Eppendorf, Hamburg, Germany) with an in situ PCR adapter and incubating it at 40 °C for 20 min. Then 120 μl of RT–PCR reaction mix was loaded by placing it on the dry array and centrifuging the array for 5 min at 3,000 r.p.m. at 4 °C (Beckman Coulter,). With tweezers, a PCR adhesive (TSS-RTQ-100, Excel Scientific Inc., Victorville, CA) was manually cut to have the same footprint as the microwell array and placed on top of the microwell array (by submerging it in the mix). Then the gasket was slowly removed, and the whole array was spun for 10 min at 3,000 r.p.m. in a plate centrifuge (Allegra 6KR, Beckman Coulter, Concord, MA, USA) at 4 °C. The sealed array was then rinsed with di-H 2 O and gently dried with nitrogen. A 20 × 20 × 0.15 mm cover glass slide (VWR International Inc., USA) was placed on top of the array and secured with PCR adhesive tape (Excel Scientific). Mineral oil (M8662, Sigma-Aldrich, St Lois, MO, USA) was then placed between the cover slide and the microscope slide to prevent any evaporation during the thermal cycling. Thermocycling was performed by placing the loaded and sealed microarray on the Eppendorf Mastercycler Gradient (Eppendorf, Hamburg, Germany) with the in situ PCR adapter. RT–PCR amplification A Lux primer/probe set (FAM labelled Lux primers 100M-01, Invitrogen, Carlsbad, CA, USA) with a FAM fluorophore for the mouse housekeeping gene GapDH was used for the BB88/HL60 cell mix detection. For the BB88/HL60 discrimination, the AmpliGrid Single Cell One-Step RT–PCR (Single Cell One-Step RT–PCR System AmpliGrid, Advalytix, Beckman Coulter, Munich, Germany) reaction mix was used according to the manufacturer’s instructions and prepared to a total mix of 120 μl with a final primer/probe concentration of 0.2 μM. The reaction mix was loaded in the microwell array and sealed as described in the ‘Cell preparation and loading’ section above. Mineral oil (M8662, Sigma-Aldrich) was added to improve the heat conductivity between the device and the cycler. The thermocycling profile used was as recommended by the manufacturer: 42 °C for 10 min, 50 °C for 10 min, 58 °C for 30 min, 95 °C for 10 min; followed by 30 cycles of 94 °C for 30 s, 60 °C for 60 s, 72 °C for 60 s. The reaction finalized with 72 °C for 10 min. Generally there were some dry wells at the edges of the well array at the end of the reaction. Off chip reactions were performed with the same reaction mix but were loaded into conventional 384 well plates (Applied Biosystems, Warrington, UK) with a reaction volume of 5 μl and cycled in a conventional real time machine (7900HT Fast Real time PCR System, Applied Biosystems, Warrington, UK). RT–PCR reactions of pAW109 RNA were performed by loading the microwells with a known number of RNA targets obtained from the GeneAmp RNA PCR controls kit (cat # 4308238, Life Technologies, Foster City, CA, USA) and reverse transcribed into cDNA and PCR amplified using the primer set for pAW109 RNA included in the kit. Fluorescence signal was achieved by adding 20 × Evagreen dye from Biotium (Hayward, CA, USA) to the RT–PCR mix. The RT–PCR master mix consisted of 16.5 μl 2 × Reaction Mix (CellsDirect, PN 46-7200, Invitrogen, USA), 0.75 μl SuperScript III RT Platinum Taq Mix (CellsDirect, PN 46-7200, Invitrogen, USA), 1.5 μl 20x Evagreen, 1.5 μl of pAW109 forward and reveres primers (GeneAmp RNA PCR controls kit, cat # 4308238, Life Technologies, Foster City, CA, USA), 5.25 μl of DEPC-treated water (CellsDirect, PN 46-7200, Invitrogen, USA) and 3 μl of pAW109 RNA. The thermo-cycling profile used was 55 °C for 45 min, 95 °C for 6 min; followed by 12 cycles of 95 °C for 60 s, 65 °C for 60 s, and 18 cycles of 95 °C for 60 s, 60 °C for 60 s and finally held at 4 °C until the chip was scanned. RT–PCR reactions for the detection of Birc6, Itga2b, Slamf1, Cyr61, Camp, Dntt, Bcl11b and Itgam were performed in multiplex with mouse Beta Actin by mixing 66.6 μl 2x Reaction Mix (CellsDirect, PN 46-7200, Invitrogen, USA), 3 μl SuperScript III RT Platinum Taq Mix (CellsDirect, PN 46-7200, Invitrogen, USA), 6 μl 20x Beta Actin assay mix with a Cy5 Taqman probe ( mActB RTprimerDB ID: 2846, PrimeTime Std qPCR Assay, IDT Integrated DNA Technologies, San Diego CA, USA), 39 ul of DEPC-treated water (CellsDirect, PN 46-7200, Invitrogen, USA) and 6 μl 20x assay mix with a FAM Taqman probe for the gene of interest. The table below lists the assay mixes used. All assay mixes include multi-exon spanning primers to prevent the amplification of DNA. All primers were purchased from IDT Integrated DNA Technologies. The thermocycling profile used was 55 °C for 45 min, 95 °C for 6 min; followed by 12 cycles of 95 °C for 60 s, 65 °C for 60 s and 18 cycles of 95 °C for 60 s, 60 °C for 60 s and finally held at 4 °C until the chip was scanned. PCR amplification Amplification of genomic DNA was done using the 2x Power SYBR(R) Green PCR Mater Mix (Applied Biosystems). The mix was prepared according to the manufacturer’s instructions with a forward and reverse primer final concentration of 0.2 μM, BB88 cell concentration of 500 cells per μl and a total volume of 60 μl. The thermocycling programme was 95 °C for 10 min, followed by 40 cycles of 94 °C for 30 s and 60 °C for 1 min. The forward and reverse primers were designed to amplify the Nanog promoter region and had the following sequences: Nanog forward primer—5′-TTGGGACCAGCTAGAGCAAT-3′; Nanog Reverse primer—5′-CCAGGCTTGTCTACCACCAT-3′; The reaction mix was loaded in the microwell array and sealed as describe in the ‘Cell preparation and loading’ section above. Off-chip reactions were performed with the same reaction mix but were loaded into conventional 384-well plates (Applied Biosystems) with a reaction volume of 5 μl and cycled in a conventional real time machine (7900HT Fast Real-time PCR System, Applied Biosystems). Microscopy For experiments that did not require full array imaging, manual imaging was used. The array of microwells was manually imaged in three locations per array on an epifluorescent microscope (DM 4000B, Leica Microsystems GmbH, Wetzlar, Germany) at × 10 magnification (Objective Floutar 10x/0.3, Leica Microsystems GmbH). Excitation light sources were produced with a xenon lamp and passed through a quad-band filter set for specific excitation bandwidths. Images were captured using a Retiga 2000R digital camera (QImaging, Canada). The capture was controlled using the ImagePro 6.3 software (Media Cybernetics). Brightfield, FITC and Cy5 fluorescent images were captured. Full array imaging was achieved by placing the array on an automatic slide scanning system, Zeiss AxioImager DIC/Fluorescence Microscope (Neuroscience Microscopy Service, Stanford, CA, USA). One hundred and eight, 0% overlap regions of the array were imaged at × 10. Each location was imaged for DIC, FITC (Zeiss Filter Set 38HE: FITC/eGFP/Alexa 488) and Cy5 (Zeiss Filter Set 50: Cy5/Alexa647) fluorescence. The exposure was set to cover 70% of the dynamic range of the CCD (Peltier cooled, Sony ICX 285 sensor). Cell labelling for counting Cells were first washed once with PBS, then resuspended in 1 ml PBS with 1 μl of the labelling dye (Evagreen, Life Technologies, Carlsbad, CA, USA). Labelling was carried out at room temperature for 30 min. The cells were washed two times with PBS and then counted using a haemocytometer (Bright-Line, Hausser Scientific, Horsham, PA, USA) and re-suspended at the desired concentration and loaded on the microwell array. Image analysis and plotting Captured images were analysed using custom scripts in ImageJ v4.4 (NIH, USA) and MatLAB 5.3 (MathWorks, El Segundo CA, USA) software. A detailed description of the algorithms used to extract the data from the images is shown in the flow chart in Fig. 4 . In brief, using ImageJ, the global background was subtracted from each fluorescent image. Then using differential interference contrast (DIC) images, the location of each microwell was established; using the Cy5 images, the location of each cell was established. The mean florescence of each micro-well was quantified with the MatLAB script after removing pixels that belonged to the cell within the well. The mean fluorescence surrounding the well was also subtracted from the mean fluorescence of the well; thus, the fluorescence was normalized across the array. Using the Cy5 quantification to calculate the threshold fluorescence, the wells without cells were identified and discarded from the plot. The mean intensity of the empty wells was used to normalize the fluorescence signal. All plotting of the density scatter plots was performed using custom scripts within MatLAB. Heterogeneity likelihood calculation To test whether gene expression values for a particular gene were heterogeneous as represented by a bimodal or multi-component distribution, we used the StepMiner statistic [31] and recomputed the null distribution from randomly generated data. We defined the statistic as (SSTO–SSE)/SSE, where SSTO is the sum of the square error from the average and SSE, the fitted best step [31] . To compute a null distribution of this statistic, we generated the same number of values from a normal random distribution. We computed the HLS as (1−( P -value)), where the P -value (see Supplementary Figs 9 and 10 ) equals to the probability of the corresponding statistic exceeding the statistic from the original data. Sample size calculation The sample size calculations were generated using numeric Monter Carlo simulations through a custom script written in Matlab 2010b. A Gaussian mixture model was assumed and implemented based on a random number generator using the Matlab normrnd function. Then different sizes of random samples were taken from a two-component Gaussian mixture model with varying parameters. The random samples were used as input into a variational Bayesian inference algorithm [37] for detecting the number of components that make up the Gaussian mixture. The random simulations were iteratively repeated until the mean of the statistical power reached a 95% confidence interval of less than 0.1 for each parameter configuration. From these simulations, the probability of correct component number estimation was calculated and plotted ( Fig. 1b ) for the different sample sizes. How to cite this article: Dimov, I. K. et al. Discriminating cellular heterogeneity using microwell-based RNA cytometry. Nat. Commun. 5:3451 doi: 10.1038/ncomms4451 (2014).